Impact of genomic polymorphisms on the repertoire of human MHC class I-associated peptides For decades, the global impact of genomic polymorphisms on the repertoire of peptides presented by major histocompatibility complex (MHC) has remained a matter of speculation. Here we present a novel approach that enables high-throughput discovery of polymorphic MHC class I-associated peptides (MIPs), which play a major role in allorecognition. On the basis of comprehensive analyses of the genomic landscape of MIPs eluted from B lymphoblasts of two MHC-identical siblings, we show that 0.5% of non-synonymous single nucleotide variations are represented in the MIP repertoire. The 34 polymorphic MIPs found in our subjects are encoded by bi-allelic loci with dominant and recessive alleles. Our analyses show that, at the population level, 12% of the MIP-coding exome is polymorphic. Our method provides fundamental insights into the relationship between the genomic self and the immune self and accelerates the discovery of polymorphic MIPs (also known as minor histocompatibility antigens). Classic adaptive CD8 T cells recognize major histocompatibility complex (MHC) class I-associated peptides (MIPs), and the ensemble of MIPs presented on the surface of a cell (the ‘immunopeptidome’) establishes its immunologic identity [1] , [2] , [3] . CD8 T cells are eminently self-referential and highly discriminant: they are selected on self-MIPs, sustained by self-MIPs and must swiftly react when confronted with non-self-MIPs interspersed in a sea of self-MIPs [4] , [5] . Understanding the molecular definition of self for CD8 T cells has been made possible by high-throughput mass spectrometry (MS) analyses of MIPs [6] , [7] , [8] , [9] , [10] , [11] , [12] . Progress in this field has been heralded by the development of MS instruments whose sensitivity, dynamic range and mass accuracy are orders of magnitude superior to those of analysers available a decade ago [13] . High-throughput MS studies have revealed that the immunopeptidome is highly complex and that its composition (that is, the source of MIPs) cannot be inferred solely from transcript or protein abundance [7] , [9] , [12] , [14] , [15] , [16] . The MHC I region contains two major classes of genes: modern classical MHC Ia genes (for example, HLA-A , HLA-B and HLA-C in humans) and more ancient MHC Ib genes (for example, HLA-E and HLA-G ). MHC Ia molecules play a dominant role in adaptive immunity. They bind MIPs and are encoded by the most polymorphic genes known [17] , [18] . Since MHC Ia allotypes display distinct peptide-binding motifs, the HLA (human leukocyte antigen) genotype has a major impact on the MIP repertoire [19] . Notably, almost all genetic polymorphisms in HLA Ia alleles are located in exons 2 and 3, which encode the MIP-binding pocket. Besides, the 1,000 Genomes Project Consortium has identified 38 million single nucleotide polymorphisms (SNP), 1.4 million short insertions and deletions, after comprehensive studies on 1,092 subjects [18] . This raises the fundamental question: what might be the impact of the numerous polymorphisms outside the MHC on the MIP repertoire? In other words, to what extent do genomic polymorphisms translate into differences in the immunopeptidome? Several MIPs have been found to derive from polymorphic genomic regions [20] , [21] . For historical reasons, these polymorphic MIPs are referred to as minor histocompatibility antigens (MiHAs). MiHAs are essentially genetic polymorphisms viewed from a T-cell perspective. MiHA-coding alleles can be dominant or recessive at the peptide level. Thus, a non-synonymous SNP (ns-SNP) in an MIP-coding genomic sequence will either hinder MIP generation (recessive allele) or generate a variant MIP (dominant allele) [22] , [23] , [24] . MiHAs are generally defined according to three criteria: they are present in some but not in all subjects bearing a given HLA allele, their presence/absence is linked to a well-defined genetic polymorphism and they can elicit allo-immune T-cell responses [22] , [23] , [24] . Three decades of research have led to the discovery of about 35 human MiHAs encoded by autosomes and presented by HLA class I molecules [23] , [24] . The discovery of each MiHA has been a major endeavour, if not a technical tour de force [25] , [26] , [27] , [28] , [29] , [30] . However, owing to the lack of a suitable systems-level approach, we ignore the global impact of non-MHC genomic polymorphisms on the immunopeptidome (that is, what proportion of MIPs are MiHAs). On the basis of various theoretical premises, it has been speculated that the number of MiHAs expressed by an individual might be very low (less than 10) or very high (greater than 1,000) [21] , [24] . In addition to its conceptual importance, the impact of genetic polymorphisms on the immunopeptidome is of considerable medical relevance because MiHAs are the targets of three allo-immune processes: graft rejection, graft-versus-host disease and graft-versus-tumour reaction [24] , [31] , [32] , [33] , [34] , [35] , [36] . Systems-level molecular definition of the immunopeptidome can be achieved only by MS studies. However, since current MS approaches cannot reliably detect polymorphic peptides, they are inadequate for MiHA discovery [37] . Furthermore, since several steps of MIP processing cannot be modelled with available algorithms [38] , MiHA identification using prediction tools is a daunting task fraught with high false discovery rates (FDRs) [37] . To resolve this conundrum, we have developed a genoproteomic strategy that hinges on a combination of next-generation sequencing and high-throughput MS peptide identification. Our personalized platform provides unprecedented insights into the genomic landscape of human MIPs and enables high-throughput identification of MiHAs and of their underlying genomic polymorphisms. Novel approach for the identification of MIPs To evaluate the impact of non-HLA genetic polymorphisms on the MIP repertoire, we analysed the immunopeptidome of Epstein–Barr virus (EBV)-transformed B-cell lines (B-LCLs) from two non-twin HLA-identical female siblings ( Fig. 1a ). The success of our endeavour hinged on two factors: the need to reliably identify MIPs encoded by polymorphic genomic regions and to maximize the coverage of the immunopeptidome (the number of unique MIPs identified). 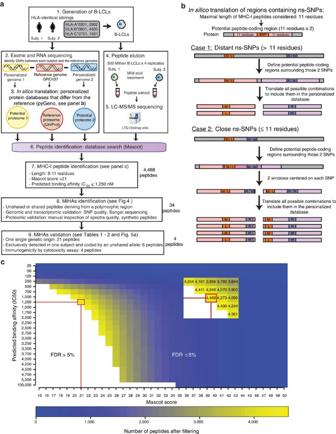Figure 1: High-throughput genoproteomic strategy used for the identification of polymorphic MIPs on B-LCLs from two HLA-identical siblings. (a) General overview of the personalized approach, which combines next-generation sequencing, MS and bioinformatics. (b) Schematic representation of the combinatorial method used to translatein silicopolymorphic regions containing ns-SNPs. (c) Combining the predicted MHC-binding affinity and Mascot score enables to discriminate between MIPs and contaminant peptides. The data set of peptides identified with an FDR≤5% was filtered according the Mascot score (which represents the confidence level of a peptide assignation), and the predicted MHC-binding affinity. The red rectangle and lines indicate the combination of values (IC50≤1,250 nM and Mascot score ≥21) that allowed identifying the maximum number of MIPs with a 5% FDR threshold. Figure 1: High-throughput genoproteomic strategy used for the identification of polymorphic MIPs on B-LCLs from two HLA-identical siblings. ( a ) General overview of the personalized approach, which combines next-generation sequencing, MS and bioinformatics. ( b ) Schematic representation of the combinatorial method used to translate in silico polymorphic regions containing ns-SNPs. ( c ) Combining the predicted MHC-binding affinity and Mascot score enables to discriminate between MIPs and contaminant peptides. The data set of peptides identified with an FDR≤5% was filtered according the Mascot score (which represents the confidence level of a peptide assignation), and the predicted MHC-binding affinity. The red rectangle and lines indicate the combination of values (IC 50 ≤1,250 nM and Mascot score ≥21) that allowed identifying the maximum number of MIPs with a 5% FDR threshold. Full size image Large-scale MS-based analyses represent the sole approach enabling comprehensive molecular definition of the MIP repertoire [1] , [12] , [39] . However, standard high-throughput MS is blind to a whole universe of polymorphic peptides. Indeed, sequencing (or assignation) of peptides by tandem MS is done using engines (for example, Mascot) that attempt to correlate tandem MS fragment ions from a sample under study with those predicted from available protein databases (for example, UniProt). Unfortunately, most polymorphic peptides are absent from these databases and tandem MS spectra from unlisted polymorphic peptides will inevitably remain unassigned or misassigned. We reasoned that the most straightforward solution to this conundrum would be to use next-generation sequencing data to create subject-specific proteomic databases that would serve as a reference for MS sequencing. Transcriptome sequencing (or RNA-seq) provides information about gene expression and can reveal sequence variation such as SNPs or RNA editing events [40] . However, lowly expressed genes might be missed by RNA-seq depending on the depth of coverage. Exome sequencing is the method of choice to capture RNA coding or exonic regions including SNPs as it tends to be less noisy than RNA-seq for variant calling and mapping [40] . Nevertheless, exome capture is limited to regions that are targeted by the probe set and not all exons are indeed transcribed in a particular cell type. Accordingly, the immunopeptidome is cell type specific [1] and preferentially derives from abundant transcripts [8] , [19] , and hence it is more likely to reflect transcriptome sequences rather than genomic sequences. To combine the benefits of both sequencing technologies and to cover as much as possible each individual’s coding genome [40] ,we sequenced both the exome and the transcriptome of B-LCLs from each subject ( Fig. 1a ). Annotated exons were covered at a depth of 130–131 × in the RNA-seq and a coverage depth of 66–158 × of exonic targets was achieved in the exome capture, with 98% of targets covered at a minimum depth of five reads ( Supplementary Data 1 ). In total, more than 53 and 50 mega base pairs of annotated exons were covered in subjects 1 and 2, representing 76–81% of the human annotated exome ( Supplementary Data 1 ). Next-generation sequencing data were used to build in silico the proteome of B-LCLs from our subjects using the in-house-developed python module pyGeno [19] ( Fig. 1b ). Following integration of exome and transcriptome sequencing, similar number of base pairs and proportions of the human exome were covered in both siblings ( Fig. 2 , track 3 blue versus orange and Supplementary Data 1 ). Exome and transcriptome sequencing data of each subject were used to identify SNPs with respect to the reference genome (GRCh37.p2, NCBI), which were then filtered according to their quality (see Methods). The majority (93.2–97.7%) of the identified SNPs are reported in the dbSNP database [41] ( Supplementary Data 2 ). SNPs were combined into a single set and integrated at their respective position on the reference human genome to obtain two ‘personalized genomes’, from which we extracted and translated every transcript (see Methods section). The translations were then compiled in two ‘personalized protein databases’, one for each subject. 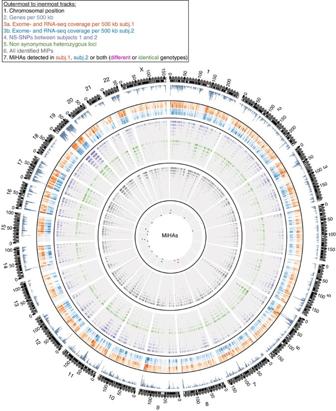Figure 2: Integrative view of the genomic landscape of the MIP repertoire of HLA-identical siblings. Circos plot showing similar proportions of sequenced genomic and transcriptomic regions in both siblings (tracks 1–3) and the small number of identified MiHAs (track 7) relative to the number of MS-detected MIPs (track 6) and sequenced polymorphic regions (tracks 4–5). From outermost to innermost tracks: (1) ideogram indicating chromosomal positions for each chromosome, (2) histogram depicting the number of genes for 500 kb windows, (3) heat map showing the fraction of bases of 500 kb windows covered by exome (outer circle) or transcriptome (inner circle) sequencing of subjects 1 (orange) and 2 (blue), (4) tile graph of 4,833 ns-SNP between siblings (purple), (5) tile graph of 3,774 heterozygous loci where both alleles are shared by the two subjects and lead to non-synonymous amino-acid changes (green), (6) tile graph representing genomic regions that give rise to 4,468 MIPs, (7) each dot represents one single gene-encoded MiHA deriving from regions containing ns-SNPs and detected by MS in subjects 1 (orange), 2 (blue) or both (green). Figure 2: Integrative view of the genomic landscape of the MIP repertoire of HLA-identical siblings. Circos plot showing similar proportions of sequenced genomic and transcriptomic regions in both siblings (tracks 1–3) and the small number of identified MiHAs (track 7) relative to the number of MS-detected MIPs (track 6) and sequenced polymorphic regions (tracks 4–5). From outermost to innermost tracks: (1) ideogram indicating chromosomal positions for each chromosome, (2) histogram depicting the number of genes for 500 kb windows, (3) heat map showing the fraction of bases of 500 kb windows covered by exome (outer circle) or transcriptome (inner circle) sequencing of subjects 1 (orange) and 2 (blue), (4) tile graph of 4,833 ns-SNP between siblings (purple), (5) tile graph of 3,774 heterozygous loci where both alleles are shared by the two subjects and lead to non-synonymous amino-acid changes (green), (6) tile graph representing genomic regions that give rise to 4,468 MIPs, (7) each dot represents one single gene-encoded MiHA deriving from regions containing ns-SNPs and detected by MS in subjects 1 (orange), 2 (blue) or both (green). Full size image MIPs were eluted from the cell surface by mild acid elution performed on four biological replicates of 500 million cells for each subject. Eluted peptides were desalted and separated on strong cation exchange chromatography before liquid chromatography–tandem mass spectrometry (LC–MS/MS) analyses using high-resolution precursor and product ion spectra. Compared with other methods such as MHC I immunoprecipitation, acid elution has the advantage of harvesting almost all MIPs, irrespective of their MHC-binding affinity [42] . However, direct acid elution can increase the amount of non-MHC contaminant peptides that are recovered [8] . To maximize the sensitivity and specificity of MIP detection, we have therefore developed an analysis pipeline that relies on a combination of four parameters: (i) the canonical MIP length of 8–11 amino acids, (ii) the predicted MHC-binding affinity given by the NetMHCcons algorithm [43] , (iii) the Mascot score, which reflects the quality of peptide assignation and (iv) the FDR, which indicates the proportion of decoy (false) versus target (true) identifications (see Methods section). We found that for an FDR of 5%, the best coverage of the immunopeptidome was obtained by combining a Mascot score ≥21 and an MHC-binding affinity ≤1,250 nM ( Fig. 1c and Supplementary Figs 1 and 2 ). Next, we compared the number of peptide identifications obtained by Mascot using the regular human protein database (UniProt) and personalized databases based on exome and transcriptome sequencing ( Supplementary Fig. 3a ). We identified 4,468 unique MIPs from the two personalized databases ( Supplementary Data 3 ). The numbers of MIPs identified with the reference database versus personalized databases were similar with a 96% overlap ( Supplementary Fig. 3a ). Notably, replacement of reference with the personalized databases had no impact on the quality (Mascot score) of identified peptides ( Supplementary Fig. 3b ). The MIP repertoire of HLA-identical siblings We have previously shown that the HLA genotype has a major impact on the MIP repertoire of MHC-mismatched individuals [19] . Here we compared the MIP repertoire of HLA-identical siblings to evaluate the impact of non-HLA genetic polymorphisms on the immunopeptidome. In addition to having identical HLA genotypes, the two siblings showed similar expression levels of the HLA-A , HLA - B and HLA - C genes ( Supplementary Data 4 ) and of the total amount of MHC class I molecules at the cell surface ( Supplementary Fig. 4 ). Following mild acid elution of peptides of comparable efficacy between subjects ( Supplementary Fig. 4 ), we identified a total of 4,468 MIPs encoded by genes from all chromosomes ( Fig. 2 , track 6 and Supplementary Data 3 ), detected in a variable number of biological replicates ( Fig. 3a ) and associated to HLA-A*03:01, -A*29:02, -B*08:01, -B*44:03 or –C*16:01. Similar numbers of MIPs were identified from the two subjects (4,114 in subject 1 and 4,186 in subject 2). As expected, the majority of the MIPs (86%) were detected in both subjects ( Fig. 3a ). Most MIPs (75%) had a predicted binding affinity <500 nM ( Fig. 3b ). We found no significant difference in the average binding affinity of 282 peptides exclusively detected in subject 1 versus 351 peptides exclusively detected in subject 2 ( Fig. 3b ). Furthermore, the number of peptides predicted to bind each of the HLA molecules was similar between the two subjects, suggesting that both siblings had comparable surface expression of each of the five HLA allelic products tested ( Fig. 3c ). Collectively, these results show that the MIP repertoire of HLA-identical subjects is similar yet not identical. 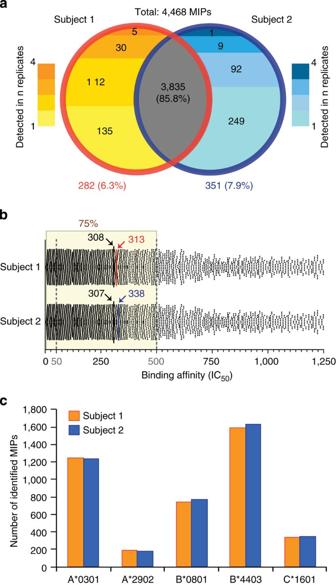Figure 3: HLA-identical siblings present similar but not identical MIP repertoires. (a) Venn diagram showing that 86% of MIPs from HLA-identical siblings were detected in both subjects. A total of 4,468 MIPs were identified in the siblings after analysis of eight biological samples (four biological replicates per sibling). MIPs were detected in variable number of biological replicates. For peptides exclusively detected in one subject, the number of replicates in which the peptide was found is shown. The total numbers of MIPs exclusively detected in subject 1 or 2 are shown in red and blue, respectively. (b) Scatter plot showing that 75% of identified MIPs are predicted to bind their respective HLA molecules with an IC50<500 nM. The IC50for five HLA alleles was calculated with the NetMHCcons algorithm. For each peptide (represented by dots), the best binding score for a specific allele was kept. The yellow box highlights 75% of all peptides. The black lines and values indicate the average binding affinity of all peptides identified in each sibling. Red and blue lines and numbers represent the average binding affinity of 282 and 351 unshared peptides exclusively detected in subject 1 or 2, respectively. The predicted binding affinity of the two sets of unshared MIPs was statistically indistinguishable (P=8.5 × 106by two-tailed Mann–Whitney test). (c) The number of peptides associated with each HLA molecule was similar between the two subjects. Figure 3: HLA-identical siblings present similar but not identical MIP repertoires. ( a ) Venn diagram showing that 86% of MIPs from HLA-identical siblings were detected in both subjects. A total of 4,468 MIPs were identified in the siblings after analysis of eight biological samples (four biological replicates per sibling). MIPs were detected in variable number of biological replicates. For peptides exclusively detected in one subject, the number of replicates in which the peptide was found is shown. The total numbers of MIPs exclusively detected in subject 1 or 2 are shown in red and blue, respectively. ( b ) Scatter plot showing that 75% of identified MIPs are predicted to bind their respective HLA molecules with an IC 50 <500 nM. The IC 50 for five HLA alleles was calculated with the NetMHCcons algorithm. For each peptide (represented by dots), the best binding score for a specific allele was kept. The yellow box highlights 75% of all peptides. The black lines and values indicate the average binding affinity of all peptides identified in each sibling. Red and blue lines and numbers represent the average binding affinity of 282 and 351 unshared peptides exclusively detected in subject 1 or 2, respectively. The predicted binding affinity of the two sets of unshared MIPs was statistically indistinguishable ( P= 8.5 × 10 6 by two-tailed Mann–Whitney test). ( c ) The number of peptides associated with each HLA molecule was similar between the two subjects. Full size image MiHAs among MIPs detected exclusively in one subject MiHAs are typically encoded by bi-allelic loci [22] , [23] . For each locus where two alleles are present in our subjects, three genotypes are possible: AA, AB and BB. At the peptidomic level, each allele can be dominant (generate a MIP) or recessive (a null allele that generates no MIP). Moreover, by comparing MIPs eluted from two HLA-identical individuals, dominant MiHAs can be separated into two groups based on their MS detection: shared MIPs and MIPs detected exclusively in one subject. MIPs detected in only one subject derive from different genotypes (for example, AA versus BB and AA versus A B if only B is a dominant allele), while shared MIPs can originate from identical genotypes (AB versus AB) or from different genotypes (for example, BB versus A B if only B is a dominant allele). Thus, subjects can be similar at the peptidomic level (display shared MIPs), although they have different genotypes ( Fig. 4 ). 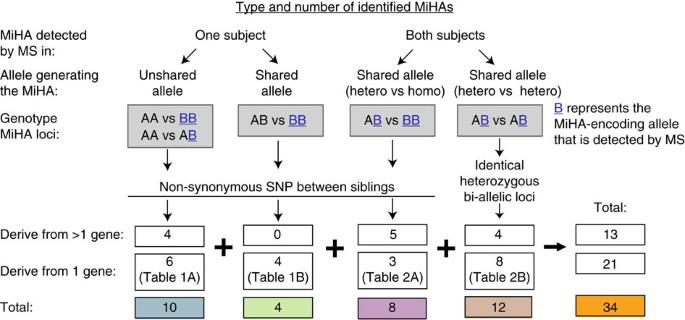Figure 4: Overview of MiHAs identified following analysis of genomic and peptidomic data from our two subjects. Identified MiHAs were classified according to the genotype of MiHA-encoding loci, the presence of the allele generating the MiHA in one or both siblings, their genetic origin (one or multiple genes) and the detection of the MiHA by MS. The total number of identified MiHAs is shown for each category. Figure 4: Overview of MiHAs identified following analysis of genomic and peptidomic data from our two subjects. Identified MiHAs were classified according to the genotype of MiHA-encoding loci, the presence of the allele generating the MiHA in one or both siblings, their genetic origin (one or multiple genes) and the detection of the MiHA by MS. The total number of identified MiHAs is shown for each category. Full size image In our search for MiHAs, we first performed in-depth analyses of MIPs detected in only one subject ( Fig. 3a ). Here the key finding was that out of 633 MIPs exclusively detected in one subject, only 14 (2%) were encoded by genomic regions harbouring ns-SNPs between the two subjects ( Fig. 4 , n =10+4 and Supplementary Data 3 ). The origin of 4 of these 14 MIPs was ambiguous (they could derive from several genes), whereas the other 10 MiHAs were assigned to a single gene ( Fig. 4 , n =6+4 and Table 1 ). The genetic polymorphisms responsible for almost all MiHAs corresponded to reported SNPs ( Table 1 ). Consistent with previous findings on human MiHAs [23] , only one of the two possible variants was detected by MS for each MiHA locus ( Table 1 ). In other words, at the peptide level, one allele was dominant (generated a MIP) and one was recessive (generated no MIP; Table 1 ). In 5 out of 10 cases, absence of the variant MiHA at the cell surface could be explained by a decreased binding affinity of the variant for the corresponding HLA molecule (IC 50 difference≥2 × ). Nine of our best characterized MiHAs are novel, whereas one (KEFED G IINW) corresponds to the allelic variant of a previously reported MiHA (KEFED D IINW) [44] that has been recently identified [45] . Four MiHAs were exclusively detected by MS in one of the subjects, although they derived from a shared allele ( Table 1B and Fig. 4 ). In all cases, the MiHA was detected in the subject homozygous for the corresponding allele but not in the heterozygous subject ( Table 1 ). This suggests that zygosity influences MiHA abundance and that low abundance MiHAs may fall below the MS detection threshold in heterozygous subjects. Consistent with this, the MS intensity for these four MiHAs was low in the homozygous subject ( Supplementary Data 3 ). Six MiHAs were coded by an allele present only in one subject ( Table 1A ), and were thus potentially immunogenic for the other sibling. We further validated the peptide sequence using MS/MS from their respective synthetic peptide ( Supplementary Fig. 5a ). Furthermore, we confirmed the presence of the ns-SNP in the corresponding DNA and/or complementary DNA regions of these six MiHAs in both subjects by Sanger sequencing ( Supplementary Fig. 6 ). Then, we determined the immunogenicity of four of these MiHAs by cytotoxicity assays. Peripheral blood mononuclear cells (PBMCs) from the MIP-negative subject were stimulated with autologous dendritic cells (DCs) pulsed with an unshared MIP detected in the other subject. Primed cells were restimulated with autologous B-LCLs pulsed with the same peptide, and then tested for in vitro cytotoxicity activity against autologous B-LCLs (MIP-negative) and allogeneic B-LCLs (MIP-positive). In all cases, in vitro- generated MiHA-specific cytotoxic T lymphocytes selectively killed allogeneic MiHA-positive B-LCLs but not autologous MiHA-negative B-LCLs ( Fig. 5a ). Table 1 MiHAs detected by MS in only one of the two subjects and resulting from ns-SNPs in MIP-coding regions. 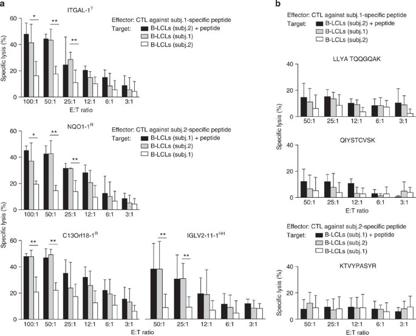Figure 5: Only polymorphic MIPs are immunogenic. Frozen PBMCs from the MIP-negative subject were thawed and stimulated with autologous DCs pulsed with an unshared MIP detected in the other individual. Primed cells were restimulated with irradiated autologous B-LCLs pulsed with the same peptide for another 7 days. Restimulated cells were tested forin vitrocytotoxicity activity against autologous B-LCLs pulsed with the relevant peptide (positive control, black), unpulsed autologous B-LCLs (negative control, white) or MIP-positive allogeneic B-LCLs (test, grey) at various effector-to-target (E:T) ratios. The minimal cytotoxic activity against unpulsed autologous B-LCLs is most probably because of recognition of EBV epitopes. Average and s.d. of three or four independent experiments are shown. Significant differences are indicated by *P<0.05 or **P<0.01, two-tailed Student’st-test. (a) MIPs encoded by polymorphic loci and detected exclusively in one subject. (b) MIPs encoded by non-polymorphic loci but detected exclusively in one subject. Full size table Figure 5: Only polymorphic MIPs are immunogenic. Frozen PBMCs from the MIP-negative subject were thawed and stimulated with autologous DCs pulsed with an unshared MIP detected in the other individual. Primed cells were restimulated with irradiated autologous B-LCLs pulsed with the same peptide for another 7 days. Restimulated cells were tested for in vitro cytotoxicity activity against autologous B-LCLs pulsed with the relevant peptide (positive control, black), unpulsed autologous B-LCLs (negative control, white) or MIP-positive allogeneic B-LCLs (test, grey) at various effector-to-target (E:T) ratios. The minimal cytotoxic activity against unpulsed autologous B-LCLs is most probably because of recognition of EBV epitopes. Average and s.d. of three or four independent experiments are shown. Significant differences are indicated by * P <0.05 or ** P <0.01, two-tailed Student’s t -test. ( a ) MIPs encoded by polymorphic loci and detected exclusively in one subject. ( b ) MIPs encoded by non-polymorphic loci but detected exclusively in one subject. Full size image We next sought to determine why some MIPs derived from non-polymorphic regions were detected by MS in only one subject ( n =633−14=619; Fig. 3a ). Could they be MiHAs whose presence is regulated by cis - or trans -acting polymorphisms (outside the MIP-coding genomic sequence) that would affect MIP processing [22] , [24] ? The MS/MS spectra of each of these MIPs were manually validated and, to further confirm the absence of the MIPs in one of the two subjects, we searched these MIPs in two additional biological replicates from each cell line. Most non-polymorphic MIPs found in only one subject were detected in only one or two replicates ( Fig. 3a ). This suggests that the presence of these MIPs was inconsistent, perhaps reflecting in part the limited sensitivity of MS. However, 41 unshared MIPs could not be discarded so easily because they were detected in three to six replicates of one sibling and absent in six replicates of the other sibling. With the exception of two cases, exclusive detection of these MIPs in one of the siblings was not caused by interindividual differences in abundance of the MIP source transcript ( Supplementary Fig. 7a ) or in the expression of the MIP-coding exon ( Supplementary Fig. 7b ), nor by differences in the expression of genes involved in the antigen processing and presentation pathway ( Supplementary Data 4 ). We therefore selected for further analyses the three most enticing MIPs coded by non-polymorphic regions but detected by MS in only one subject: MIPs showing the best values for the predicted binding affinity, MS intensity, reproducibility and Mascot score ( Supplementary Data 3 ). We further confirmed their absence in one of the subjects by comparing the corresponding extracted ion chromatograms ( Supplementary Fig. 5b ) and validated their MS/MS spectra with synthetic peptides ( Supplementary Fig. 5c ). We reasoned that if these MIPs were MiHAs, they should be immunogenic, even if their presence was dictated by unidentified polymorphisms outside the MIP-coding genomic sequence. None of the tested MIPs could elicit the generation of cytotoxic T cells in the MIP-negative sibling ( Fig. 5b ). We therefore failed to discover a single MiHA among MIPs coded by non-polymorphic regions. The most parsimonious explanation is that these MIPs were simply differentially expressed peptides whose abundance was below the MS detection threshold in B-LCLs from one subject. A plausible explanation would be that exclusive detection of these MIPs in one subject reflects cellular differences caused by EBV infection during the establishment of the B-LCLs and/or clonal variation [46] . Accordingly, we conclude that identification of MiHAs absolutely requires a combination of MS and genomic data. Reliance solely on MS detection would overestimate the number of MiHAs. In contrast, the use of personalized databases based on whole exome and transcriptome sequencing allows to rapidly identifying genuine MiHAs coded by polymorphic loci. The global imprint of ns-SNPs on the MIP repertoire To assess the global imprint of ns-SNPs on the MIP repertoire, we asked the question: what proportion of ns-SNPs between our two subjects were located in MIP-coding exomic sequences? By comparing the combination of whole exome and RNA-seq data from our two subjects, we found a total of 4,833 ns-SNPs, 87% of which are reported as ‘validated’ in dbSNP ( Fig. 2 , track 4 and Supplementary Data 2 ). Overall, 26 of these ns-SNPs were located in regions coding for 22 MiHAs identified by MS, of which 13 originated from a single gene ( Fig. 4 , n =6+4+3) and are depicted in the Circos plot ( Fig. 2 , track 4 versus 7 blue, orange and pink) and 9 have an ambiguous origin ( Fig. 4 , n =4+0+5 and Supplementary Data 3 ). The 13 unambiguously assigned MiHAs were exclusively detected ( Table 1 ) or shared ( Table 2A ) at the peptidomic level. Thus, from a genomic perspective, only 0.5% of all ns-SNPs (26/4,833) found between our subjects were represented in their MIP repertoire. Table 2 MiHAs detected in both subjects and coded by loci harbouring ns-SNPs. Full size table Identification of MiHAs among shared MIPs Among 3,835 shared MIPs ( Fig. 3a ), 20 were encoded by bi-allelic loci and therefore represent MiHAs ( Fig. 4 , n =8+12). These shared MIPs would not be immunogenic for our subjects but would be immunogenic for subjects homozygous for the alternative allele. In eight cases, one subject was homozygous for a dominant MiHA allele (AA) and the other subject was heterozygous for the dominant and a recessive allele (AB; Fig. 4 ). The origin of five of these eight MiHAs was ambiguous (they could derive from several genes), whereas the other three MiHAs were assigned to a single gene ( Fig. 4 and Table 2 ). The exome of our subjects shared 3,774 heterozygous loci ( Fig. 2 , track 5). Twelve MiHAs derived from such bi-allelic loci for which our subjects shared the same heterozygous genotype (AB). Eight of these 12 MiHAs could be unambiguously assigned to a single gene ( Fig. 2 , track 7 in green, Fig. 4 and Table 2B ). The two alleles were co-dominant in one case, whereas only one allele was dominant (identified by MS) in the other cases. Notably, in four of the shared MiHAs, the product of the recessive allele was predicted to have a lower MHC-binding affinity than the product of the dominant allele ( Table 2 ). Differences in the MIP repertoire of HLA-identical siblings Comparison of genomic and proteomic data from our subjects led to the discovery of 34 MiHAs ( Fig. 4 ), of which 21 were unambiguously assigned to a specific gene ( Fig. 2 , track 7 and Tables 1 and 2 ). Out of 34 MiHAs, 14 were found in only one of the two subjects, whereas 20 MiHAs were shared MIPs ( Fig. 4 ). Without considering the 4 MiHAs that were exclusively detected in one subject but that derived from a shared allele ( Table 1B ), this means that out of 4,468 MIPs only 10 (0.22%) would be immunogenic for one of our subjects. Assuming that non-polymorphic MIPs detected exclusively in one subject are not immunogenic ( Fig. 5b ), this means that each subject would be tolerant to about 99.8% of the MIPs found on the B-LCLs of this sibling. The use of personalized databases for tandem MS sequencing was instrumental in the discovery of many MiHAs. Eleven of the 21 MiHAs listed in Tables 1 and 2 would have been missed in the absence of personalized databases, because these 11 peptides were absent in the Uniprot database. Polymorphic MIP-coding regions at the population level We searched in the dbSNP database for validated ns-SNPs in the genomic sequences coding our 4,468 MIPs. We found that at the population level, 88% of our MIP-coding sequences were invariant, whereas 12% contained at least one ns-SNP: 670 ns-SNPs were found in the genomic region coding for 536 MIPs ( Fig. 6a,b and Supplementary Data 5 ). Hence, at the population level, 536 MiHAs can be presented by the five HLA class I molecules studied herein: HLA-A*03:01, -A*29:02, -B*08:01, -B*44:03 and -C*16:01. Further studies will be required to determine the number of dominant and recessive peptide variants encoded by these 536 MiHA loci. 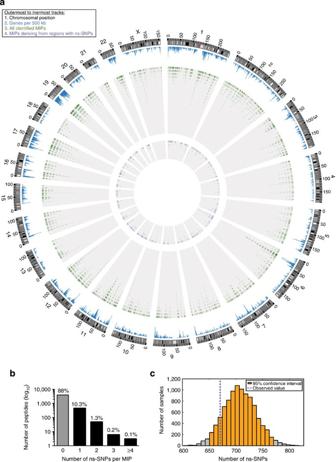Figure 6: Frequency of ns-SNPs in the MIP-coding exome. (a) Circos plot illustrates the relative proportion of polymorphic MIPs (n=536) in the immunopeptidome and the genomic location of their coding loci. (b) Histogram showing the number and percentages of MIP-coding regions containing ns-SNPs in the global population. We used dbSNP to find validated ns-SNPs in the exomic sequences encoding the 4,468 MIPs identified in our subjects. In the case of MIPs deriving from multiple source regions, the average number of ns-SNPs of all possible MIP source regions was calculated. (c) The 4,468 MIPs of our subjects were encoded by 13,404 nucleotides. We performed 10,000 random samplings of 4,468 exomic sequences (containing a total of 13,404 nucleotides) from the human reference exome (Ensemble GRCh37.65). In all samplings, the frequency of exomic sequences coding for 8-,9-,10- and 11-mers was identical to the frequency found in the 4,468 MIP-coding sequences from our subjects. The histogram depicts the distribution of validated ns-SNPs (dbSNP) in exomic sequences from the global population found in 10,000 random samplings of the whole exome. The average number of ns-SNPs of all random samplings was 708 (s.d.: 30.4, 95% confidence interval: 650–768 shown in orange). The blue dotted line shows the number of ns-SNPs (n=670) in the exomic sequences coding for the MIPs detected in our subjects. Figure 6: Frequency of ns-SNPs in the MIP-coding exome. ( a ) Circos plot illustrates the relative proportion of polymorphic MIPs ( n =536) in the immunopeptidome and the genomic location of their coding loci. ( b ) Histogram showing the number and percentages of MIP-coding regions containing ns-SNPs in the global population. We used dbSNP to find validated ns-SNPs in the exomic sequences encoding the 4,468 MIPs identified in our subjects. In the case of MIPs deriving from multiple source regions, the average number of ns-SNPs of all possible MIP source regions was calculated. ( c ) The 4,468 MIPs of our subjects were encoded by 13,404 nucleotides. We performed 10,000 random samplings of 4,468 exomic sequences (containing a total of 13,404 nucleotides) from the human reference exome (Ensemble GRCh37.65). In all samplings, the frequency of exomic sequences coding for 8-,9-,10- and 11-mers was identical to the frequency found in the 4,468 MIP-coding sequences from our subjects. The histogram depicts the distribution of validated ns-SNPs (dbSNP) in exomic sequences from the global population found in 10,000 random samplings of the whole exome. The average number of ns-SNPs of all random samplings was 708 (s.d. : 30.4, 95% confidence interval: 650–768 shown in orange). The blue dotted line shows the number of ns-SNPs ( n =670) in the exomic sequences coding for the MIPs detected in our subjects. Full size image Bias in favour or against ns-SNPs in MIP-coding regions We next wished to compare, in the global population, the frequency of ns-SNPs in the whole exome versus the frequency in the 4,468 exomic sequences coding for the MIPs identified herein. To this end, we designed a bootstrap procedure (10,000 iterations) based on random samplings of 4,468 peptide-coding regions (13,404 base pairs/sampling) from the human reference exome (Ensemble GRCh37.65). For each sampling, we then calculated the number of validated ns-SNPs reported in dbSNP ( Fig. 6c ). Each sampling contained the same proportion of exomic sequences coding for 8-,9-,10- and 11-mers as the MIP-coding sequences from our subjects. We found that the number of ns-SNPs in the MIP-coding exome ( n =670) fell in the range of ns-SNPs found in 10,000 random samplings of the whole exome (average=708; 95% confidence interval=650–768). We therefore conclude that the MIP-coding exome reflects the frequency of ns-SNPs in the whole human exome. MS is the sole method that enables direct identification of MIPs and large-scale analyses of the MIP repertoire [1] , [15] . Indirect predictions based on reverse immunology approaches are fraught with FDRs that may reach 95% [47] , [48] . Currently, MS sequencing has been largely limited to peptides represented in the reference UniProt database. Our work demonstrates that the universe of peptides identified by MS can be expanded and refined by using personalized databases that include whole exome and transcriptome sequencing data. As well stated by Princiotta et al. ‘Despite the fact that quantitative aspects of systems are critical to their understanding, they are frequently ignored’ [49] . In line with this concept, our data provide the answer to a longstanding question: what is the proportion of invariant versus polymorphic MIPs presented by MHC molecules? In other words, to what extent do non-MHC genomic polymorphisms enhance the interindividual variability of the immunopeptidome? We found that, at the population level, at least one ns-SNP is found in 12% of exomic sequences coding the MIPs presented by five common HLA class I allotypes. That about 88% of the genomic landscape of the MHC class I immunopeptidome is invariant in the global population illustrates the overwhelming importance of the HLA genotype in defining the content of the MHC class I immunopeptidome. In-depth analyses of genomic and proteomic data revealed that about 0.5% of ns-SNPs between the exome of our subjects were represented in their MIP repertoire. Consequently, 10 MIPs coded by an unshared allele were unique to one subject and might elicit allogeneic T-cell responses from his sibling, as demonstrated for four of them. Integration of personalized genomic and proteomic data was absolutely essential for identification of these rare polymorphic MIPs interspersed among thousands of non-polymorphic MIPs. Since the MIP repertoire is moulded by the transcriptome, some MIPs are ubiquitous and others are cell lineage specific [8] , [50] . Accordingly, various cell types present non-identical MIP repertoires. MIPs derive mostly from transcripts expressed at medium to high levels (as opposed to very low or low levels), and about 8,500 transcripts are expressed at medium to high levels in B-LCLs [19] . We therefore posit that, at the organismal level, the total number of MiHAs derived from unshared ns-SNPs between two HLA-identical siblings would be about 2.5-fold the number found in B cells, assuming a total number of 21,000 human transcripts (that is, 10 × (21,000/8,500)=25). Unrelated individuals share fewer gene sequences than siblings. As a consequence, it has been calculated that the frequency of unshared MiHAs is increased by about 1.8-fold in unrelated (HLA-matched) subjects relative to siblings [23] . Thus, two unrelated HLA-identical subjects would display about 45 unshared MHC class I-restricted MiHAs. Of note, these numbers might increase with better sequencing coverage of difficult regions (for example, GC-rich) and more sensitive MS instruments. As illustrated here, four low abundance MiHAs could only be detected in the homozygous but not in the heterozygous individual. Furthermore, our estimate could vary depending on the cell type and it does not take into account MiHAs presented by MHC class II proteins. Although only six MHC class II-restricted MiHAs have been discovered in humans [24] , [51] , a fair estimate of their repertoire will require systems-level studies using methods such as the one described herein. All MHC antigens are dominant. Our data show that this is not the case for MiHAs. With a single exception, all MiHA loci had one dominant (MIP generating) and one recessive (no MIP generated) allele ( Tables 1 and 2 ). This observation is clearly consistent with population analyses of 10 well-characterized autosomal MiHA loci: only one locus has two dominant alleles [23] . For slightly less than 50% of our recessive alleles, the absence of MIP could be explained by a decreased MHC-binding affinity of peptides. For the other recessive alleles, the absence of MIP must be due to interference of the polymorphism with some step in MIP processing that precedes MHC binding (for example, cleavage by the proteasome or other proteases) [3] , [38] . With tens of thousands of proteins, mammalian cells are the most complex entity in the antigenic universe faced by our immune system [52] . Theoretical estimates suggest that the immunopeptidome contains 0.1% of the 9-mer sequences present in the proteome [1] . Few peptides win the fierce competition for inclusion in the immunopeptidome. Thus, if we consider MiHAs coded by dominant alleles as winners, it follows that in most cases a single ns-SNP is sufficient to transform winners into losers (the recessive alleles). This is an eloquent reminder that we cannot predict the molecular composition of the immunopeptidome based on our limited understanding of the complexity of the MIP processing pathway. Allogeneic haematopoietic cell transplantation has led to the discovery of the allogeneic graft-versus-leukemia effect, which remains the most widely effective strategy for cancer immunotherapy in humans. The graft-versus-leukemia effect is mediated mainly, if not exclusively, by donor T cells that recognize host MiHAs. In line with recent progress in the field of cell therapy, MiHAs are therefore attractive targets for adoptive T-cell immunotherapy of cancer, particularly haematologic cancers [31] , [32] , [33] , [34] , [35] , [36] . However, because of the low number of molecularly defined human MiHAs, less than 30% of patients would currently be eligible for immunotherapy targeted to specific MiHAs [53] . Our report reveals a strategy for high-throughput MiHA discovery that could greatly accelerate the development of MiHA-targeted immunotherapy. Our genoproteomic method combining next-generation sequencing and MS shows how it is possible to accurately identify by MS any MIP, provided that its source DNA or RNA has been sequenced. The personalized protein databases could be further refined by including other types of polymorphisms such as indels and using linkage disequilibrium information to diminish the number of possible proteins that will be expressed in an individual, given his SNPs. This approach opens new avenues in systems immunology and should be invaluable for exploration of several ‘black holes’ in the immunopeptidome. One particularly important black hole is the ‘cancer immunome’ [54] . Compelling evidence suggests that the most immunogenic antigens present on cancer cells are mutant peptides derived from the numerous mutations found in neoplastic cells [55] , [56] , [57] . However, tumour-specific mutant peptides (alike MiHAs) are not detected by standard large-scale MS approaches. We posit that our method should enable discovery of tumour-specific peptides (the product of somatic mutations) with the same accuracy as MiHAs (the product of germline genetic polymorphisms). Accordingly, our next priority will be to use this method to explore the impact of the cancer mutations on the immunopeptidome of cancer cells. Cell culture and HLA typing This study was approved by the Comité d’Éthique de la Recherche de l’Hôpital Maisonneuve-Rosemont and all subjects provided written informed consent. As fresh blood samples were required for cytotoxicity assays, we elected to generate new B-LCLs from available donors, instead of studying the highly characterized B-LCLs from the Centre d'Etude du Polymorphisme Humain. PBMCs were isolated from blood samples of two non-twin HLA-identical Caucasian female siblings (54 and 56 years old). B-LCLs were derived from PBMCs with Ficoll-Paque Plus (Amersham) followed by EBV infection as described [58] . Ten million PBMCs in 2.5 ml complete RPMI-10 medium were incubated with 1 ml EBV (strain B95-8) suspension as obtained from the supplier (ATCC VR-1492) for 2 h in a 37 °C water bath. Complete RPMI-10 containing 1 μ ml −1 of cyclosporine A (Sigma-Aldrich) was added to the cell suspension for a total volume of 10 ml) and incubated for 3–5 weeks in a humidified 37 °C, 5% CO 2 incubator. High-resolution HLA genotyping was performed at the Maisonneuve-Rosemont Hospital. The two siblings are HLA-A*03:01,*29:02; B*08:01,*44:03; C*07:01,*16:01; DRB1*03:01,*07:01. RNA extraction and preparation of transcriptome libraries Total RNA was isolated from 5 million B-LCLs using RNeasy mini kit including DNase I treatment (Qiagen) according to the manufacturer’s instructions. Total RNA was quantified using the NanoDrop 2000 (Thermo Scientific) and RNA quality was assessed with the 2100 Bioanalyzer (Agilent Technologies). Transcriptome libraries were generated from 1 μg of total RNA using the TruSeq RNA Sample Preparation Kit v2 (Illumina) following the manufacturer’s protocol. In brief, poly-A messenger RNA was purified using poly-T oligo-attached magnetic beads using two rounds of purification. During the second elution of the poly-A RNA, the RNA was fragmented and primed for cDNA synthesis. Reverse transcription of the first strand was performed using random primers and SuperScript II (Invitrogen). A second round of reverse transcription was done to generate a double-stranded cDNA, which was then purified using Agencourt AMpure XP PCR purification system (Beckman Coulter). End repair of fragmented cDNA, adenylation of the 3′ ends and ligation of adaptors were completed following the manufacturer’s protocol. Enrichment of DNA fragments containing adapter molecules on both ends was done using 15 cycles of PCR amplification and the Illumina PCR mix and primers cocktail. DNA extraction and exome capture Genomic DNA was extracted from 5 million B-LCLs using the PureLink Genomic DNA Mini Kit (Invitrogen) according to the manufacturer’s instructions. DNA was quantified and quality assessed using the NanoDrop 2000 (Thermo Scientific). Genomic libraries were constructed from 1 μg of genomic DNA using the TruSeq DNA Sample Preparation Kit (v2) (Illumina) following the manufacturer’s protocol. We used 500 ng of DNA-Seq libraries for hybrid selection-based exome enrichment with the TruSeq exome enrichment kit (Illumina) according to the manufacturer’s instructions. Sequencing and mapping of whole transcriptome and exome Paired-end (2 × 100 bp) sequencing was performed using the Illumina HiSeq2000 machine running TruSeq v3 chemistry. Two RNA-Seq or four exomic libraries were sequenced per lane (eight lanes per slide). Cluster density was targeted at around 600–800 k clusters mm −1 (ref. 2 ). The Illumina chastity quality filter was used to remove the low-quality reads. The chastity of a base call is the ratio of the intensity of the greatest signal divided by the sum of the two greatest signals. Reads passed this filter if no more than one base call in the first 25 cycles had a chastity <0.6. More than 96% of the reads passed this filter ( Supplementary Data 1 ). Sequence data were mapped to the human reference genome (hg19) using the Casava 1.8.1 and the Eland v2e mapping softwares (Illumina). First, the *.bcl files were converted into compressed FASTQ files, followed by demultiplexing of separate multiplexed sequence runs by index. Single reads were aligned to the human reference genome using the multiseed and gapped alignment method. Multiseed alignment works by aligning the first seed of 32 bases and consecutive seeds separately. Gapped alignment extends each candidate alignment to the full length of the read and allows for gaps up to 10 bases. The following criteria were applied: (i) a read contains at least one seed that matches with at most two mismatches without gaps and (ii) gaps were allowed for the whole read, as long as they correct at least five mismatches downstream. For each candidate alignment, a probability score, which is based on the sequencing base quality values and the positions of the mismatches, was calculated. The alignment score of a read, which is expressed on the Phred scale, was computed from the probability scores of the candidate alignments. The best alignment for a given read corresponded to the candidate alignment with the highest probability score and was kept if the alignment score exceeded a threshold. Read alignments were further filtered out if they contained adjacent insertion/deletion events or if paired-end anomalies were present. Reads that mapped at two or more locations were not included in further analyses. For the exome paired-end libraries, the best scoring alignments for each half of the pair were computed and compared to find the best paired-read alignments according to the estimated insert size distribution. In the case of RNA-seq libraries, an additional alignment was performed against splice junctions and contaminants (mitochondrial and ribosomal RNA). Sequences mapping to contaminants were discarded, whereas reads uniquely mapping to splice junctions were kept and converted back to genome coordinates. Quantification of transcript expression We used two methods to estimate and compare transcript expression between subjects. In the first method, the Casava 1.8.1 software (Illumina) was used to estimate gene or exon expression levels (RNA-seq) measured as read per kilobases of exon model per million mapped reads using the following formula: gene or exon RPKM=10 9 × Cb/Nb × L , where Cb is the number of bases that fall on the feature, Nb is the total number of mapped bases and L is the length of the feature in base pairs. We also used the DESeq package [59] , which is based on raw counts, to compare transcript expression. Transcript expression level was not considered in SNP calling. Identification of SNPs and read counting Variant call, indel detection and read counting were done using the Casava 1.8.1 software (Illumina). Reads were re-aligned around candidate indels to improve the quality of variant calls and site coverage summaries. Individual base calls were further filtered based on mismatch density or ambiguity and the remaining base calls were used to predict site genotypes. Casava was also used to retrieve all SNPs observed between the reference genome (GRCh37.p2, NCBI) and the sequenced transcriptome and exome of our subjects. SNPs and indel calls near centromeres and within high copy-number regions were removed. For each called SNP, Casava calculates the most probable genotype (max_gt) and a Q -value expressing the probability of the most probable genotype (Qmax_gt). The Q -value is a quality score that measures the probability that a base is called incorrectly and was used to filter out low-quality SNPs (see ‘ In silico- generated proteomes and personalized databases’ section). SNPs sequenced with at least 5 × coverage were kept. This information (.txt files) was loaded into an in-house python module, pyGeno [19] , for further processing. In silico- generated proteomes and personalized databases We used various in-house scripts that rely on pyGeno for data retrieval, parsing and processing. We integrated the exome sequencing data to the transcriptome sequencing data. For every SNP found by transcriptome sequencing, we retained the most probable genotype if the Q -value (Qmax_gt) was ≥20, which corresponds to a 1% error rate (a higher quality score indicates a smaller probability of error). If the SNP was also covered by the exome sequencing, we included not only the most probable genotype found by RNA-seq but also all bases in common with the exome sequencing. We also included the genotypes of SNPs that were only found by exome sequencing and that had a Q -value ≥20. Finally, we included all bases of SNPs called by both the transcriptome and exome sequencing regardless of the Q -value. The retained genotypes of all SNPs were then integrated in the reference genome (GRCh37.p2, fasta file) at their right position to construct a ‘personalized genome’ for each subject. These personalized genomes were used to extract all transcripts reported in the Ensembl gene set (GRCh37.65, gtf file) for all chromosomes except for the Y chromosome and mitochondrial DNA. These transcripts were then in silico translated into proteins using the reading frame specified in the Ensembl gene set. Considering that the vast majority of MIPs have a maximum length of 11 amino acids, we established a window of 21 amino acids centred at each heterozygous ns-SNP. When a window contained more than one SNP, we translated in silico all possible combinations and included them in the personalized databases ( Fig. 1b ). Finally, we compiled all translation products into two fasta file databases (one for each subject) that were used for the identification of MIPs (see ‘MS/MS sequencing and peptide clustering’ section). Both resulting databases had a similar size, in terms of number of residues (36,007,210 in subject 1 and 36,010,026 in subject 2) and number of entries (95,806 in subject 1 and 95,687 in subject 2). Moreover, their size is comparable to the size of the reference UniProt human database used (43,384,120 residues and 75,530 entries). MS/MS sequencing and peptide clustering On the basis of our previous studies on MS data reproducibility across technical and biological replicates [8] , we prepared four biological replicates of 5 × 10 8 exponentially growing B-LCLs from each subject. MIPs were released by mild acid treatment, desalted on an HLB cartridge 30 cc, filtered with a 3,000-Da cutoff membrane and separated into seven fractions by cation exchange chromatography using an off-line 1,100 series binary LC system (Agilent Technologies) as previously described [8] , [9] . Fractions containing MIPs were resuspended in 0.2% formic acid and analysed by LC–MS/MS using an Eksigent LC system coupled to a LTQ-Orbitrap ELITE mass spectrometer (Thermo Electron). Peptides were separated on a custom C 18 reversed phase column (150 μm i.d. X 100 mm, Jupiter Proteo 4 μm, Phenomenex) using a flow rate of 600 nl min −1 and a linear gradient of 3–60% aqueous ACN (0.2% formic acid) in 120 min. Full mass spectra were acquired with the Orbitrap analyser operated at a resolving power of 30,000 (at m / z 400). Mass calibration used an internal lock mass (protonated (Si(CH 3 ) 2 O)) 6 ; m/z 445.120029) and mass accuracy of peptide measurements was within 5 p.p.m. MS/MS spectra were acquired at higher energy collisional dissociation with a normalized collision energy of 35%. Up to six precursor ions were accumulated to a target value of 50,000 with a maximum injection time of 300 ms and fragment ions were transferred to the Orbitrap analyser operating at a resolution of 15,000 at m/z 400. Mass spectra were analysed using Xcalibur software and peak lists were generated using Mascot distiller Version 2.3.2 ( http://www.matrixscience.com ). Database searches were performed against UniProt Human database (43,384,120 residues, released on 2 April 2013), databases specific to subjects 1 and 2 (34,976,580 and 34,990,381 residues, respectively, see ‘ in silico- generated proteome and personalized databases’ section) and EBV_B95.8 database (40,946 residues), using Mascot (Version 2.3.2, Matrix Science). To calculate the FDR, we performed a Mascot search against a concatenated target/decoy database using the human UniProt or subject-specific databases. The target represents the forward sequences and the decoy its reverse counterparts. Mass tolerances for precursor and fragment ions were set to 5 p.p.m. and 0.02 Da, respectively. Searches were performed without enzyme specificity with variable modifications for cysteinylation, phosphorylation (Ser, Thr and Tyr), oxidation (Met) and deamidation (Asn, Gln). Raw data files were converted to peptide maps comprising m/z values, charge state, retention time and intensity for all detected ions above a threshold of 8,000 counts using in-house software (Proteoprofile) [9] . Peptide maps corresponding to all identified peptide ions were aligned together to correlate their abundances across sample sets and replicates. The MS/MS spectra of MIPs detected exclusively in one subject were validated manually. Identification of MIPs MIP identification was based on four criteria: (i) the canonical MIP length of 8–11 amino acids, (ii) the predicted MHC-binding affinity given by the NetMHCcons algorithm [43] , (iii) the Mascot score, which reflects the quality of peptide assignation, and (iv) the FDR, which indicates the proportion of decoy (false) versus target (true) identifications. First, we evaluated the correlation between these parameters. We found a strong correlation (0.88) between FDR values <60% and MHC-binding affinity values ≤1,750 nM for all 8–11-mers ( Supplementary Fig. 1 ). Indeed, the proportion of peptides with an MHC-binding affinity ≤1,750 nM increases as the FDR decreases ( Supplementary Fig. 2a ). This correlation was specific to MIPs, since no correlation was found for random peptides ( Supplementary Figs 1 and 2b ). These results show that low FDR values allow enrichment of high-affinity peptides (MHC-binding affinity ≤1,750 nM) and thus of MIPs. However, the drawback of using a stringent low FDR as the main filter is that the total number of identifications considerably decreases ( Supplementary Fig. 2a ) as well as the proportion of small peptides (8–9-mers) identified ( Supplementary Fig. 2c ). Accordingly, the relative proportion of peptides found in target versus decoy decreased with increasing peptide length [60] , in accordance with the notion that short peptides such as MIPs generally require higher Mascot scores to achieve a low FDR. Moreover, the tandem MS fragment ions of MIPs are less predictable and evenly distributed than those of tryptic peptides that further complicate their assignment by database search engines such as Mascot. To set a more suitable Mascot score threshold for high-throughput MIP detection, we evaluated the relationship between the Mascot score and the predicted binding affinity for all 8–11-mer peptides identified with an FDR≤5% ( Fig. 1c ). Then, we calculated the number of MIPs identified with all combinations of Mascot score and predicted binding affinity. We found that the highest number of MIP identifications was obtained by combining a Mascot score ≥21 and an MHC-binding affinity ≤1,250 nM at a 5% FDR ( Fig. 1c ). MS/MS validation of a subset of MIPs Polymorphic and non-polymorphic MIPs exclusively detected in one of the two subjects ( Table 1 and Supplementary Data 3 ) were synthesized by Bio Basic Inc. and JPT peptide technologies. Subsequently, 500 fmols of each peptide were injected in the LTQ-Orbitrap ELITE mass spectrometer using the same parameters as those used to analyse the biological samples. Ns-SNPs found in MIP-coding regions in the population For each MIP, we retrieved the coordinates of the peptide-coding DNA region. These coordinates were then used to extract both the corresponding reference sequence and all non-synonymous validated SNPs reported by dbSNP (Build 137) for that region. For MIPs deriving from multiple source regions, the number of ns-SNPs reported corresponds to that of the MIP source region possessing the maximal number of ns-SNPs. Random peptide sampling We constructed a genome-wide index. To do so, we indexed every coding sequences reported in the Ensembl gene set (GRCh37.65), except for those located in the Y chromosome or the mitochondrial DNA, into a segment tree. Next, we kept only the first layer of the tree and removed the gaps between the indexed regions, effectively transforming the tree into a coding DNA sequence list, which was used for the random peptide sampling. For each of the 4,468 identified peptides, a random peptide of the same length and that fell entirely into a single coding DNA sequence, was chosen. Next, for each randomly selected peptide, we counted the number of ns-SNPs reported in dbSNP137 (validated and missense). The distribution was obtained after repeating the sampling of 4,468 random peptides 10,000 times. PCR and Sanger sequencing PCR amplification of the MiHA-encoding DNA and cDNA regions was performed with the Phusion High-Fidelity PCR kit (New England BioLabs). For each candidate, 1–2 pairs of sequencing primers were designed manually and with the PrimerQuest software (Integrated DNA Technologies, Supplementary Table 1 ), and were synthesized by Sigma. PCR products were purified with the PureLink Quick Gel Extraction Kit (Invitrogen). Sanger sequencing was performed on candidate DNA and cDNA at the IRIC’s Genomics Platform. Sequencing results were visualized with the Sequencher software v4.7 (Gene Codes Corporation). Cytotoxicity assays DCs were generated from frozen PBMCs, as previously described [61] . To generate cytotoxic T cells, autologous DCs were irradiated (4,000 cGy), loaded with 2 μM of peptide and cultured for 7 days with freshly thawed autologous PBMCs at a DC:T-cell ratio of 1:10. From day 7, responder T cells were restimulated for seven additional days with irradiated autologous B-LCLs pulsed with the same peptide (B-LCL:T-cell ratio 1:5). Expanding T cells were cultured in RPMI 1,640 (Invitrogen) containing 10% human serum (Sigma-Aldrich) and L -glutamine. IL-2 (50 U ml −1 ) was added for the last 5 days of the culture. Cytotoxicity assays were performed as described [9] , with minor modifications. In brief, B-LCLs were labelled with carboxyfluorescein succinimidyl ester (CFSE; Invitrogen), extensively washed, irradiated (4,000 cGy) and then used as targets in cytotoxicity assays. Target cells were plated in 96-well U-bottom plates at 5,000 cells per well. Effector cells were added at different effector-to-target ratios in a final volume of 200 μl per well. Plates were centrifuged and incubated for 18–20 h at 37 °C. Flow cytometry analysis was performed using a LSRII cytometer with a high-throughput sampler device (BD Biosciences). The percentage of specific lysis was calculated as follows: [(number of CFSE + cells remaining after incubation with unpulsed target cells−number of CFSE + cells remaining after incubation with peptide-pulsed target cells)/number of CFSE + cells remaining after incubation with unpulsed target cells] × 100. Statistical analysis and data visualization The two-tailed Student’s t -test was used to identify differentially expressed MIPs and MiHAs that induced cytotoxicity. The two-tailed Mann–Whitney test was used to compare the MHC-binding affinity of MIPs detected exclusively in one subject. Differentially expressed transcripts were identified with the DESeq package that uses a model based on the negative binomial distribution [59] . The Spearman correlation was used to evaluate the relationship between differences in MIP abundance and differences in MIP-coding gene or exon expression. The genomic location of identified MIPs including MiHAs and the RNA-seq and exome sequencing coverage were visualized with the Circos software [62] . The Integrative Genomics Viewer v2.0 (ref. 63 ) was used to visualize and inspect regions coding MIPs including MiHAs. Accession codes: MIP MS/MS spectra data were deposited in the PeptideAtlas database (PeptideAtlas, http://www.peptideatlas.org/ ) under accession code PASS00270. MHC-I peptide sequences were deposited in the Immune Epitope Database ( http://www.iedb.org/ ) under submission code 1000565. RNA-seq data were deposited in the Gene Expression Omnibus database ( http://www.ncbi.nlm.nih.gov/geo/ ) under accession code GSE48918 , Exome data were deposited in the NCBI Sequence Read Archive ( http://www.ncbi.nlm.nih.gov/sra ) under accession code PRJNA210790. How to cite this article: Granados, D. P. et al. Impact of genomic polymorphisms on the repertoire of human MHC class I-associated peptides. Nat. Commun. 5:3600 doi: 10.1038/ncomms4600 (2014).